Quasi-monoenergetic laser-plasma acceleration of electrons to 2 GeV Laser-plasma accelerators of only a centimetre’s length have produced nearly monoenergetic electron bunches with energy as high as 1 GeV. Scaling these compact accelerators to multi-gigaelectronvolt energy would open the prospect of building X-ray free-electron lasers and linear colliders hundreds of times smaller than conventional facilities, but the 1 GeV barrier has so far proven insurmountable. Here, by applying new petawatt laser technology, we produce electron bunches with a spectrum prominently peaked at 2 GeV with only a few per cent energy spread and unprecedented sub-milliradian divergence. Petawatt pulses inject ambient plasma electrons into the laser-driven accelerator at much lower density than was previously possible, thereby overcoming the principal physical barriers to multi-gigaelectronvolt acceleration: dephasing between laser-driven wake and accelerating electrons and laser pulse erosion. Simulations indicate that with improvements in the laser-pulse focus quality, acceleration to nearly 10 GeV should be possible with the available pulse energy. Since the first cyclotrons, betatrons and linear accelerators were developed in the 1930s, particle accelerators have evolved into the twenty first century’s most powerful scientific instruments in fields ranging from fundamental physics to molecular biology, to medicine [1] . However, their size and expense now threaten the future of teraelectronvolt-class accelerator research, exemplified by the recent discovery of a Higgs-like boson [2] , and inhibit wide availability of gigaelectronvolt (GeV)-class accelerators that underlie coherent X-ray sources used for biological, chemical and condensed matter research. In 1979, Tajima and Dawson [3] proposed the idea of accelerating charged particles by surfing them on electron density waves propagating through underdense plasma in the wake of an intense ultrashort laser pulse. Such plasma wakes sustain electric fields of gigavolts per centimetre (GV cm −1 ), thousands of times above the electric breakdown threshold of conventional accelerators, thus opening the possibility of miniature accelerators. Two decades of experiments, enabled by wide availability of terawatt (TW) femtosecond (fs) lasers starting in the 1990s, have yielded laser-plasma accelerators (LPAs) of millimetre-to-centimetre length [4] that capture and accelerate ambient plasma electrons quasi-monoenergetically to energy as high as 1 GeV [5] , with tails reaching 1.4 GeV [6] , and with angular divergence as small as a few milliradian. These experiments were restricted to plasma electron densities n e >10 18 cm −3 at which TW laser pulses could resonantly excite a wake and inject [7] plasma electrons into it. However, at those densities the maximum electron energy is inherently limited to ~1 GeV by dephasing between accelerating electrons and plasma wake, and by erosion of the laser pulse by the plasma [8] . The quest for multi-GeV LPAs is motivated by the possibility of constructing compact linear colliders [9] for future high-energy physics research and table-top sources of ultrashort, coherent hard X-rays [10] for physical, chemical and biological studies of dynamics at the atomic scale. From computer simulations, certain general requirements for multi-GeV LPAs are well known. First, as for sub-GeV accelerators the LPA should operate in a ‘blowout’ regime—that is, one in which the laser pulse is strong enough to blow out electrons to form an electron density ‘bubble’ [8] , [11] . Both numerical modelling [8] , [11] and experimental diagnostics [12] have shown that bubble formation is essential for producing collimated, quasi-monoenergetic electron beams. Second, plasma density must be reduced to n e <10 18 cm −3 to increase dephasing length L D and pump-depletion length L PD to multiple centimetres, factors that more than compensate for the slightly weaker accelerating field at lower density. Third, laser peak power P must be kept well above the critical power GW for relativistic self focusing. Here ω 0 is the laser frequency and is the plasma frequency. This enables the drive pulse to self focus and self compress during its initial non-linear interaction with the plasma, increasing its intensity to a level at which blowout occurs, and helps it to self guide over multiple Rayleigh lengths once acceleration begins, thereby exploiting the increased acceleration length set by L D and L PD . For n e in the low 10 17 cm −3 range, P must therefore approach ~10 15 W, or 1 petawatt ( PW), a capability that is just emerging from recent advances in laser technology. Although these basic requirements are quantitatively understood, theory and simulation are less precise in predicting self injection of plasma electrons into the bubble at n e <10 18 cm −3 , a property that greatly simplifies accelerator design by eliminating the need for an external injector. Although some simulations [8] and experiments [7] at n e >10 18 cm −3 have suggested scaling laws that relate self-injection threshold simply to P / P cr , these studies were restricted to an idealized ‘matched’ self-guided geometry in which the Gaussian laser pulse and plasma bubble copropagate quasi-statically. On the other hand, deviations from a matched geometry—due to the focus geometry or non-Gaussian profile (a likely feature of many first-generation PW-class laser systems) of the incident laser pulse—cause the laser pulse and bubble profiles to vary as they copropagate. Such variations profoundly affect self injection in ways not captured by simple scaling laws [13] , [14] , making self-injection thresholds difficult to predict accurately [15] . Moreover, details of bubble evolution dictate the dynamics of self injection, which in turn dictate key beam properties such as energy spread, angular divergence and background current [13] , [14] , [16] . In view of these uncertainties, previous work provides limited quantitative guidance on self-injection physics and beam properties of multi-GeV LPAs, which must therefore be discovered through laboratory experiments. Here we present the first experimental demonstration of self-injected, quasi-monoenergetic LPA of electrons well beyond 1 GeV energy. As was widely expected, this result required a PW-class laser pulse driving sub-10 18 cm −3 plasma. Our electron spectra feature a prominent narrow peak (~5% spread full width at half maximum (FWHM)) at the highest energy (a signature of bubble formation followed immediately by strong localized self injection) accompanied by a background of lower-energy electrons (a signature of continuing injection during acceleration) and by collimated ~25 keV X-rays from transverse betatron oscillations of the accelerating electrons. Our results also show that the highest electron energy (2 GeV) is achieved in a narrow range of plasma density (4 to 6 × 10 17 cm −3 ), in good agreement with simulations for our non-matched focus geometry [17] . At the same time, our results show two features not predicted by any previous simulation or scaling law. First, self-injection and multi-GeV acceleration occur despite a highly irregular focal profile. Second, the electron beam had unprecedented sub-milliradian (FWHM) divergence angle, ~4 × smaller than in previous LPA experiments, and root-mean-square (r.m.s.) pointing stability 1.4 mrad over dozens of shots. These last features, along with the quasi-monoenergetic multi-GeV spectral peak, are critical for collider and coherent light source applications. Our results were obtained with an exceptionally simple target consisting of uniform, undoped He gas, similar to the target used by Osterhoff et al. [18] , without taking advantage of specialized injection techniques [19] , [20] , [21] , [22] , preformed plasma channels [23] and structured gas cells [24] , [25] that have improved beam quality and reliability in sub-GeV LPAs. Our results thus provide a benchmark against which future multi-GeV LPAs employing such methods can be compared. 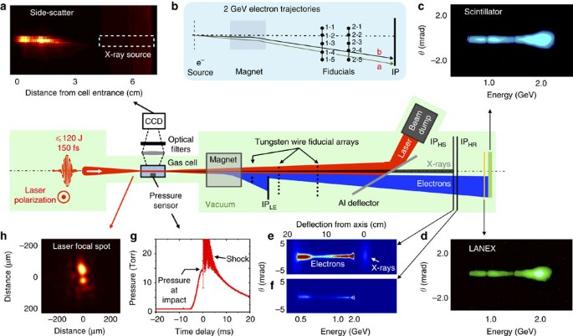Figure 1: Schematic diagram of PW laser-driven wakefield accelerator. The main components were enclosed in a vacuum chamber, highlighted in green, which was kept at 10−6Torr. The PW laser pulse, entering from the left and linearly polarized perpendicular to the plane of the drawing, was focused into the gas cell, where it created a He plasma and wake that captured and accelerated electrons to 2 GeV. Electrons and betatron X-rays emerging from the cell exit aperture passed through a magnetic field, then through two linear arrays of eight 127 μm diameter tungsten-wire fiducials located 1.256 and 1.764 m, respectively, downstream from the cell exit. A 25-μm thick Al foil deflected the transmitted laser pulse to a beam dump. Undeflected X-rays and energy-dispersed electrons above 0.5 GeV passed through this foil, and exposed in sequence a high-sensitivity (HS) imaging plate (IPHS), a high-resolution (HR) IP (IPHR), a phosphorescing screen (LANEX) and a plastic scintillator. An additional IPLErecorded low-energy (LE) electrons (<0.35 GeV) after they passed through a third array of fiducials. Surrounding panels highlight various diagnostics and details, clockwise from upper left: (a) transversely scattered light, spectrally filtered and imaged to a CCD camera (the dashed rectangle shows the region near the cell exit from which betatron X-rays originated, as determined by X-ray triangulation); (b) trajectories of 2 GeV electrons for shots that yielded the results inFig. 2a(labelled ‘a’ and ‘b’, respectively) relative to the fiducial arrays (labelled 1–1 through to 1–8 for the first array and 2–1 through to 2–8 for the second array); (c–f), unprocessed data showing electrons up to 2.3 GeV and fiducial shadows for the shot that yielded the results inFig. 2a, as detected on (c) scintillator, (d) LANEX, (e) IPHS(also showing undeflected X-rays) and (f) IPHR; (g) He pressure versus time, and an acoustic shock when the laser pulse arrived, as recorded by a fast pressure transducer; (h) a typical laser focal spot. Generation and measurement of 2 GeV electrons Figure 1 shows a schematic layout of the experiments. Linearly polarized pulses from the Texas Petawatt Laser (duration τ~ 150 fs, wavelength λ =1.057 μm, energy E laser ≤150 J) [26] were focused with f -number ( f # ) 47 into the 1.5 mm radius entrance aperture of a 7-cm-long gas cell, which was pulse-filled with 1 to 8 Torr helium (He) of 99.99% purity. Transversely scattered pump light was imaged through a side window in the cell. Accelerated electrons emerged through a 3-mm radius exit aperture and were deflected in a plane perpendicular to the laser polarization by a magnetic field from a permanent dipole magnet. This field, profiled with 1% accuracy with a Hall probe, consisted of a 4 × 4 cm central plateau surrounded by fringe fields that fell to half the plateau value within 1.2 cm of each edge and to one-tenth the plateau value within 2.5 cm. The electron beam entered the field perpendicular to one edge, aimed nominally at the centre of the plateau. The measured field deflected electrons equivalently to a uniform, fringe-free effective field of 1.10±0.01 T of 6.7 cm length. This effective field was used in calculating electron trajectories. A high-sensitivity image plate (hereafter IP HS ) detected undeflected betatron X-rays [27] , [28] , [29] and energy-dispersed electrons of energy E >0.5 GeV at the end of an evacuated tube, 2.46 m downstream from the magnet. A low-sensitivity, high-resolution IP, a phosphor (LANEX) screen and a plastic scintillator behind IP HS provided corroborating detection of GeV electrons. An additional IP detected more strongly deflected low-energy electrons (<0.35 GeV). Charge was obtained independently from different detectors based on published calibrations, yielding values that agreed within 20%. Between magnet and detectors, electrons and X-rays passed through two arrays of thin, precisely positioned tungsten-wire fiducials, which cast identifying shadows on the detectors. Triangulation based on the X-ray shadows localized the X-ray (and electron) source on each shot transversely to±75 μm along the entrance–exit aperture axis and longitudinally to ±1 cm near the cell exit. With this information, complete electron trajectories from source to detector were recovered from shadows in the electron spectrum. This enabled energy to be determined without ambiguity due to variation in launch angle θ launch [6] , [30] , [25] . Electron energy E at 2 GeV was thereby determined with ±5% uncertainty at the 2σ level (see Methods). Figure 1: Schematic diagram of PW laser-driven wakefield accelerator. The main components were enclosed in a vacuum chamber, highlighted in green, which was kept at 10 −6 Torr. The PW laser pulse, entering from the left and linearly polarized perpendicular to the plane of the drawing, was focused into the gas cell, where it created a He plasma and wake that captured and accelerated electrons to 2 GeV. Electrons and betatron X-rays emerging from the cell exit aperture passed through a magnetic field, then through two linear arrays of eight 127 μm diameter tungsten-wire fiducials located 1.256 and 1.764 m, respectively, downstream from the cell exit. A 25-μm thick Al foil deflected the transmitted laser pulse to a beam dump. Undeflected X-rays and energy-dispersed electrons above 0.5 GeV passed through this foil, and exposed in sequence a high-sensitivity (HS) imaging plate (IP HS ), a high-resolution (HR) IP (IP HR ), a phosphorescing screen (LANEX) and a plastic scintillator. An additional IP LE recorded low-energy (LE) electrons (<0.35 GeV) after they passed through a third array of fiducials. Surrounding panels highlight various diagnostics and details, clockwise from upper left: ( a ) transversely scattered light, spectrally filtered and imaged to a CCD camera (the dashed rectangle shows the region near the cell exit from which betatron X-rays originated, as determined by X-ray triangulation); ( b ) trajectories of 2 GeV electrons for shots that yielded the results in Fig. 2a (labelled ‘a’ and ‘b’, respectively) relative to the fiducial arrays (labelled 1–1 through to 1–8 for the first array and 2–1 through to 2–8 for the second array); ( c – f ), unprocessed data showing electrons up to 2.3 GeV and fiducial shadows for the shot that yielded the results in Fig. 2a , as detected on ( c ) scintillator, ( d ) LANEX, ( e ) IP HS (also showing undeflected X-rays) and ( f ) IP HR ; ( g ) He pressure versus time, and an acoustic shock when the laser pulse arrived, as recorded by a fast pressure transducer; ( h ) a typical laser focal spot. 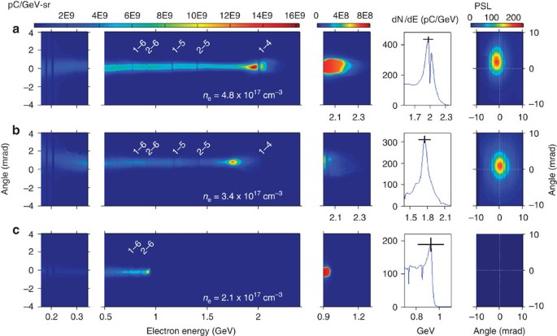Figure 2: Electron spectra and betatron X-ray profiles for three shots from the accelerator. First column: sub-GeV electron spectra recorded on IPLE; second column: GeV electron spectra recorded on IPHS; third column: detail of high-energy tails; fourth column: vertically integrated spectra around each high-energy peak; fifth column: betatron X-ray angular distribution recorded on IPHS. (a) Results for shot yielding quasi-monoenergetic peak at 2.0 GeV, withne=4.8 × 1017cm−3, obtained from raw data shown inFig. 1e. Results for (b)ne=3.4 × 1017cm−3, yielding peak at 1.8 GeV, and (c)ne=2.1 × 1017cm−3, yielding peak at 0.95 GeV.Table 1lists complete laser-plasma conditions and e-beam properties for each shot. Fiducial wire shadows are labelled as inFig. 1b. On each vertical scale, ‘0 mrad’ denotes the average vertical position of a 30-shot sequence of GeV electrons. In the fourth column, vertical error bars represent the average uncertainty in the calibration of each of IPHS, high-resolution IP (IPHR) and LANEX as charge monitors (±10%); horizontal error bars represent 2σ uncertainty in the peak position, derived from the uncertainty in fitting the calculated trajectories of electrons near 2 GeV to the observed positions of fiducial shadows on IPHSfor each shot. This uncertainty originates in turn from the combined uncertainty in fiducial wire positions (±25 μm transversely, ±2 mm longitudinally), fiducial shadow positions (±1/2 pixel, or ±50 μm), electron source position (determined by X-ray triangulation) relative to magnet and detector (±75 μm transversely, ±1 cm longitudinally) and magnetic field (±1%). Full size image Figure 2a presents electron spectra (first to fourth columns) and corresponding betatron X-ray angular distributions (fifth column) obtained from IP HS for two shots that yielded a dominant peak near E peak ~2 GeV. The laser-plasma conditions for these shots are given in the top two rows of Table 1 . Spectra recorded by other detectors corroborated the position and spectral shape of the main peaks precisely. The high-energy tails, highlighted in the third column, indicated some electrons accelerated to 2.3 GeV. Corresponding fiducial shadows in rows a–b fall at slightly different energies, because θ launch varies. Trajectories of a 2-GeV electron for shots a and b are plotted in Fig. 1b . Similar analysis for all energies established the energy scale of Fig. 2 . The main peaks near 2 GeV had angular divergence mrad (FWHM), determined from e-beam size in the vertical (v) direction (that is, transverse to the dispersion plane), 7–9 × smaller than divergence observed from GeV LPAs that relied on ionization-induced injection [6] . This signifies that electrons were injected closer to the axis of the accelerator structure in a pure He plasma than electrons injected by ionizing K -shell electrons of a high- Z dopant gas species [20] , [21] , [6] . On the other hand, when this divergence is scaled to sub-GeV electron energy, it signifies transverse electron momentum similar to that obtained in the lowest-divergence sub-GeV beams from uniform undoped gas targets (for example, 2.1±0.5 mrad FWHM at 200 MeV [18] ). Analysis of the shape of the fiducial shadows shows that divergence in the horizontal (that is, energy dispersion) plane is similar in magnitude, facilitating accurate energy analysis. In fact, the quasi-monoenergetic peaks in Fig. 2a subtend a horizontal (h) angular width (FWHM) mrad, only slightly larger than the vertical width. Thus, although the nominal width of the vertically integrated dN / dE peaks shown in the fourth column of Fig. 2a corresponds to 8–10% energy spread (FWHM), as indicated by the first number in the third column of Table 1 , the actual energy spread is considerably smaller. If we assume that vertical and horizontal angular divergences are equal, then the true energy spread of the peaks is 5–7% FWHM, as indicated parenthetically in the third column of Table 1 . This is comparable to the smallest fractional energy spread observed in sub-GeV [18] and 1 GeV [5] quasi-monoenergetic LPAs. The maximum accelerating field in the bubble regime is [8] , [24] , where is the wave-breaking field [4] and the dimensionless laser strength parameter a 0 is related to peak intensity I 0 by . For the conditions that yielded 2 GeV electrons, n e =4.8 × 10 17 cm −3 and a 0 is estimated to be ~8 after self focusing, so E z ~2 GV cm −1 . Acceleration distance is thus of the order L ~ E peak / E z , that is, 1–2 cm, if we allow for E z to be somewhat less than its maximum value. As dephasing and pump-depletion lengths ( L D ~ 20 cm; L PD ~ 10 cm) [8] exceed our gas cell length, electron energy appears to be limited primarily by the self-guiding length of the laser pulses, as discussed further below. Figure 2: Electron spectra and betatron X-ray profiles for three shots from the accelerator. First column: sub-GeV electron spectra recorded on IP LE ; second column: GeV electron spectra recorded on IP HS ; third column: detail of high-energy tails; fourth column: vertically integrated spectra around each high-energy peak; fifth column: betatron X-ray angular distribution recorded on IP HS . ( a ) Results for shot yielding quasi-monoenergetic peak at 2.0 GeV, with n e =4.8 × 10 17 cm −3 , obtained from raw data shown in Fig. 1e . Results for ( b ) n e =3.4 × 10 17 cm −3 , yielding peak at 1.8 GeV, and ( c ) n e =2.1 × 10 17 cm −3 , yielding peak at 0.95 GeV. Table 1 lists complete laser-plasma conditions and e-beam properties for each shot. Fiducial wire shadows are labelled as in Fig. 1b . On each vertical scale, ‘0 mrad’ denotes the average vertical position of a 30-shot sequence of GeV electrons. In the fourth column, vertical error bars represent the average uncertainty in the calibration of each of IP HS , high-resolution IP (IP HR ) and LANEX as charge monitors (±10%); horizontal error bars represent 2σ uncertainty in the peak position, derived from the uncertainty in fitting the calculated trajectories of electrons near 2 GeV to the observed positions of fiducial shadows on IP HS for each shot. This uncertainty originates in turn from the combined uncertainty in fiducial wire positions (±25 μm transversely, ±2 mm longitudinally), fiducial shadow positions (±1/2 pixel, or ±50 μm), electron source position (determined by X-ray triangulation) relative to magnet and detector (±75 μm transversely, ±1 cm longitudinally) and magnetic field (±1%). Full size image Table 1 Properties of and conditions for producing GeV e-beams. Full size table Figure 2c shows a typical result for similar laser parameters, but lower density ( n e =2.1 × 10 17 cm −3 ), yielding a quasi-monoenergetic ~1 GeV electron peak with negligible X-ray yield. Quasi-monoenergetic peaks, signifying bubble formation [8] , [11] , were observed at densities as low as 1.7 × 10 17 cm −3 . At lower density, self-injected electrons were observed [31] down to n e =1.0 × 10 17 cm −3 , albeit with with ~100% energy spread and energy only up to 0.3 GeV. The lower electron energy can be attributed to later injection due to weaker self focusing and to smaller accelerating fields. Electron energy dropped off for n e > 6.2 × 10 17 cm −3 , because the PW laser pulses became unstable against forward Raman scattering and filamentation [17] . Shot-to-shot consistency of the accelerator’s performance was sensitive to the position of the focal plane of the f /47 mirror. The data in Fig. 2 and the most consistent overall performance were obtained with this plane, determined by observing the focal spot of low-intensity light, within a Rayleigh range ( z R ~1.5 cm) of the gas cell entrance. Full-energy shots, however, focused ~3 cm behind this plane (that is, inside the gas cell entrance) with±2 cm r.m.s. shot-to-shot fluctuations, because of uncontrolled thermal lensing within the amplifier chain that varied from shot to shot. At this optimum mirror position determined by the low-power focus, we ran a series of ~30 shots with E laser held at 90±10 (r.m.s.) J (peak power 0.5–0.7 PW) and n e at 5.0±0.6 (r.m.s.) × 10 17 cm −3 . We observed ~GeV electrons with >90% reliability. Beam parameters and corresponding shot-to-shot r.m.s. fluctuations over this sequence were:±1.4 mrad pointing stability, 0.6±0.3 mrad angular divergence, 0.9±0.3 GeV peak energy, 50±20 pC in the peak (determined by integrating a Gaussian curve fit to the peak). The indicated pointing stability is equivalent to that of the most stable sub-GeV LPAs reported previously [18] . On the other hand, the percentage shot-to-shot fluctuations in charge (40%) and energy (33%) are larger than those of the most stable sub-GeV LPAs (for example, 16% and 2.5% r.m.s. charge and energy fluctuations, respectively, at E =200 MeV [18] ), a sign of greater fluctuations in laser-pulse focus location, focal profile and energy in our first-generation PW laser compared with more mature TW laser technology. Once the optimum low-power focus location was found during this 30-shot sequence, the 2 GeV and low n e shots in Fig. 2 were obtained during a subsequent ten-shot sequence with ~25% higher pulse energy (100< E laser <129 J) and peak power (0.6< P <0.8 PW). This trend suggests that yet higher electron energy may be obtainable with the Texas Petawatt Laser operating at its full capacity [26] of P ~1.1 PW. Electron production became intermittent when the nominal focal plane was moved > z R from the optimum location. Betatron X-rays The fifth column of Fig. 2 shows the angular distribution of betatron X-rays as recorded on IP HS . These X-rays result from the transverse wiggling motion of the accelerating electrons confined by the transverse electrostatic potential of the plasma bubble [27] , [28] , [29] , analogous to synchrotron emission from an undulator or wiggler [32] . Electrons oscillate at the betatron frequency , where γ is the continuously increasing Lorentz factor of the accelerating electrons. For betatron oscillations of small amplitude r β , and thus small strength parameter K = γr β ω β / c <<1 (undulator limit), the radiation has a narrowly peaked fundamental spectrum. For large K >>1 (wiggler limit), a broad spectrum of closely spaced harmonics peaking at a critical photon energy E crit =3 Kγ 2 ω β is emitted over a cone angle θ β ≈ K / γ . We consistently observe betatron X-rays for shots yielding at least 30 pC of electrons with at least 1 GeV energy exemplified by the shots in Fig. 2a . For these shots we observed a nearly circular X-ray profile with HWHM divergence mrad 2 , corresponding to maximum strength parameter K (v) ≈10 and K (h) ≈8.5 for the final energy E =2 GeV ( γ =4,000). This indicates that we are in the large K limit for most of the acceleration length, consistent with betatron X-rays observed from sub-GeV LPAs in the non-linear bubble regime [28] . The divergence angle of the X-rays is several times greater than that of the energetic electrons, as also observed with sub-GeV LPAs [28] . Although X-ray spectra were not measured for the shots in Fig. 2 , we estimated them for other shots that yielded >1.5 GeV electron peaks and a similar X-ray cone angle θ β by measuring X-ray transmission through aluminium and copper masks (see Fig. 3a ). 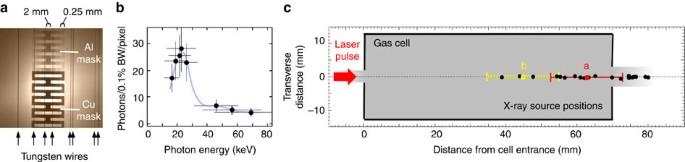Figure 3: Betatron X-ray data. (a) Typical radiograph of Al and Cu masks backlit by betatron X-rays from the accelerator recorded on IPHS. Masks vary in thickness in four lateral steps: 2 mm (centre), 1 mm, 0.5 mm and 0.25 mm (edge). Vertical lines are shadows of tungsten-wire fiducials. (b) Typical X-ray spectrum. Data points were obtained by analysing transmittance of the Cu/Al masks (see Methods). Horizontal error bars correspond to the FWHM of thefkdistribution (see Methods); vertical error bars represent uncertainty in X-ray transmission caused by scattering at edges of the filter masks, and error in reconstructing the incident X-ray intensity profile from transmission through gaps in the masks. Blue curve is a cubic spline fit to the data points. (c) X-ray source locations within the 7 cm gas cell for 22 shots that yielded >1 GeV electrons, determined by triangulation from tungsten-wire fiducial shadows. Source locations for shots inFig. 2aare labelled ‘a’ (red) and ‘b’ (yellow), respectively. Horizontal error bars (±10 mm) indicate triangulation error arising from uncertainty in measuring fiducial wire positions. Figure 3b shows a representative spectrum peaked at 25±10 keV photon energy with a tail extending beyond 70 keV extracted from mask transmission data (see Methods). This is higher than spectral peaks at ~10 keV observed from an ~0.2-GeV quasi-monoenergetic LPA [28] , but lower than peaks at >100 keV observed from an ~0.7-GeV LPA in which the betatron amplitude was resonantly enhanced by interacting with the rear of the laser pulse [29] . The X-rays observed here thus appear not to be resonantly enhanced. X-ray photon numbers range from 10 8 to 10 9 for >1.5 GeV shots (see Methods). This compares with an estimated 10 6 –10 8 photons reported from an ~0.2-GeV quasi-monoenergetic LPA [28] . Figure 3: Betatron X-ray data. ( a ) Typical radiograph of Al and Cu masks backlit by betatron X-rays from the accelerator recorded on IP HS . Masks vary in thickness in four lateral steps: 2 mm (centre), 1 mm, 0.5 mm and 0.25 mm (edge). Vertical lines are shadows of tungsten-wire fiducials. ( b ) Typical X-ray spectrum. Data points were obtained by analysing transmittance of the Cu/Al masks (see Methods). Horizontal error bars correspond to the FWHM of the f k distribution (see Methods); vertical error bars represent uncertainty in X-ray transmission caused by scattering at edges of the filter masks, and error in reconstructing the incident X-ray intensity profile from transmission through gaps in the masks. Blue curve is a cubic spline fit to the data points. ( c ) X-ray source locations within the 7 cm gas cell for 22 shots that yielded >1 GeV electrons, determined by triangulation from tungsten-wire fiducial shadows. Source locations for shots in Fig. 2a are labelled ‘a’ (red) and ‘b’ (yellow), respectively. Horizontal error bars (±10 mm) indicate triangulation error arising from uncertainty in measuring fiducial wire positions. Full size image The footprint of betatron X-rays on IP HS was wide enough to include several fiducial wire shadows. From these shadows and the corresponding wire locations, the X-ray source position was determined by simple triangulation on each shot. Figure 3c plots these source positions for over 20 shots that yielded >1 GeV electrons, including those that yielded the data in Fig. 2a (see source points labelled ‘a’ and ‘b’ in Fig. 3c ). Nearly all are concentrated within ~2 cm of the cell exit. This suggests that most laser pulses use the first ~2/3 of the gas cell to self focus to an intensity sufficient to form a plasma bubble and inject electrons into it, and the final ~1/3 of the cell to drive acceleration. We did not, however, observe any detailed correlation between the X-ray source location and the maximum electron energy. These X-ray source points were assumed to coincide with electron launch points when calculating electron trajectories through the magnet and wire fiducials. To help understand the experiment, we carried out particle-in-cell (PIC) simulations aimed at reproducing four key observations: a narrow 2 GeV peak, sub-mrad divergence, X-ray origin near the cell exit and a background of low-energy electrons. Previous PIC simulations had predicted that 100 J (200 J), 150 fs pulses focused to Gaussian spot radius w 0 ≈80 μm at the entrance of mid-10 17 cm −3 plasma would self focus, form a bubble and self inject electrons within 1.5 cm, before accelerating them quasi-monoenergetically up to 4 (7) GeV in the remaining plasma [17] . The w 0 used in these simulations was an estimate based on early Texas Petawatt Laser performance showing focused spot sizes greater than an ideal Gaussian radius ( f # λ =50 μm) or the radius of the first Airy ring of a flat-top profile (1.22 f # λ =60 μm) expected for f # =47 and λ =1.057 μm. In our experiments, incident pulse energy spread over an even larger radius w 0 ≈275 μm (white dashed circle in Fig. 4a , inset) that enclosed several ‘hotspots’, as evident in the typical high-power, equivalent-plane image of the transverse profile near the cell entrance shown in Fig. 4a , inset. A key question is whether these spots interact separately with the plasma, or merge owing to self focusing. In previous work [31] , we developed a framework for answering this question based on the non-linear Schrödinger equation (NLSE), which describes the initial laser-pulse propagation in the paraxial approximation before plasma density perturbations become important. 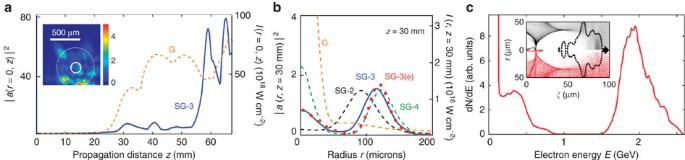Figure 4: WAKE simulation results. Initial conditions are: pre-ionized plasma of densityne=5.0 × 1017cm−3; incident laser pulse of durationτ=160 fs, energy=100 J (peak laser strength parametera0=0.58, normalized powerP/Pcr=20). (a) Laser strength parametera(r=0,z) and peak intensityI(r=0,z) along propagation axis inside plasma for initially Gaussian (G, dashed orange curve) and third-order super-Gaussian (SG-3, solid blue) pulses of radiusw0=275 μm, the latter showing two rapid self-focus/defocus cycles near the cell exit. Inset: image of incident laser profile at approximately the cell entrance, ~2 cm from its focal plane, for shot ‘a’ inFig. 2, compared with white dashed circle of radiusw0=275 μm and white solid circle of radiusw0=80 μm. Colour scale indicates intensity as a multiple of 1017W cm−2. (b) Transverse profiles atz=30 mm of initially Gaussian (G, short-dashed orange), second- (SG-2, short-dashed black), third- (SG-3, solid blue) and fourth- (SG-4, long-dashed green) order super-Gaussian pulses, showing Airy-ring-like structure for non-Gaussian profiles that is evidently critical for self injection. Each profile is plotted for the longitudinal position of maximum ∫0∞drrI(r) within the pump profile; this position differs slightly for each plot, and from the position of maximum peak intensity shown ina. For comparison, curve SG-3(φ) (red squares) shows the transverse profile atz=30 mm, calculated with the NLSE, of an initially third-order super-Gaussian multiplied by the azimuthally varying function 1+0.25(r/w0)9cos (9φ) to mimic an evolving array of hotspots. (c) Simulated electron energy spectrum atz=6.8 cm for initially third-order super-Gaussian pulse evolving as ina, showing 2 GeV peak and low-energy tail. Similar spectra were obtained for other super-Gaussian orders and for ±10% variations ina0. Inset: electron density profile, showing background plasma electrons (black, top) and test electrons (red, bottom). Injected electrons are the red feature inside evacuated bubble.ξdenotes longitudinal distance along the bubble’s axis. Black dashed curve: 8 × 1018W cm−2iso-intensity contour of laser pulse atz=6.8 cm. The NLSE has the conserved quantity [33] Figure 4: WAKE simulation results. Initial conditions are: pre-ionized plasma of density n e =5.0 × 10 17 cm −3 ; incident laser pulse of duration τ =160 fs, energy=100 J (peak laser strength parameter a 0 =0.58, normalized power P / P cr =20). ( a ) Laser strength parameter a ( r =0, z ) and peak intensity I ( r =0, z ) along propagation axis inside plasma for initially Gaussian (G, dashed orange curve) and third-order super-Gaussian (SG-3, solid blue) pulses of radius w 0 =275 μm, the latter showing two rapid self-focus/defocus cycles near the cell exit. Inset: image of incident laser profile at approximately the cell entrance, ~2 cm from its focal plane, for shot ‘a’ in Fig. 2 , compared with white dashed circle of radius w 0 =275 μm and white solid circle of radius w 0 =80 μm. Colour scale indicates intensity as a multiple of 10 17 W cm −2 . ( b ) Transverse profiles at z =30 mm of initially Gaussian (G, short-dashed orange), second- (SG-2, short-dashed black), third- (SG-3, solid blue) and fourth- (SG-4, long-dashed green) order super-Gaussian pulses, showing Airy-ring-like structure for non-Gaussian profiles that is evidently critical for self injection. Each profile is plotted for the longitudinal position of maximum ∫ 0 ∞ drrI ( r ) within the pump profile; this position differs slightly for each plot, and from the position of maximum peak intensity shown in a . For comparison, curve SG-3( φ ) (red squares) shows the transverse profile at z =30 mm, calculated with the NLSE, of an initially third-order super-Gaussian multiplied by the azimuthally varying function 1+0.25( r / w 0 ) 9 cos (9 φ ) to mimic an evolving array of hotspots. ( c ) Simulated electron energy spectrum at z =6.8 cm for initially third-order super-Gaussian pulse evolving as in a , showing 2 GeV peak and low-energy tail. Similar spectra were obtained for other super-Gaussian orders and for ±10% variations in a 0 . Inset: electron density profile, showing background plasma electrons (black, top) and test electrons (red, bottom). Injected electrons are the red feature inside evacuated bubble. ξ denotes longitudinal distance along the bubble’s axis. Black dashed curve: 8 × 10 18 W cm −2 iso-intensity contour of laser pulse at z =6.8 cm. Full size image where a ( x , t ) is the space- and time-dependent laser strength parameter. When H >0, as found previously [31] for n e =1 × 10 17 cm −3 , the hotspots propagate independently without merging. When H <0, on the other hand, as for the current experiments with higher n e , some of the hotspots merge after propagating several centimetres. We confirmed the validity of this condition using PIC simulations. As a further check, we simulated the interaction of individual hotspots with the plasma using the cylindrically symmetric PIC code WAKE [34] , modelling low-level injection with test particles. Although the stronger hotspots could often self focus and form a bubble, self injection of electrons into the accelerating structure was not observed. When the intensity of individual hotspots was increased artificially above the injection threshold, injection occurred near the cell entrance. Then, depending on the size, radial profile and energy of the hot spot it either accelerated the electrons to ~2 GeV within the first half of the cell, contradicting the X-ray source positions shown in Fig. 3c , or accelerated them well beyond 2 GeV, contradicting the observed energy spectrum. A complete understanding of the experiment thus requires that the entire irregular pulse profile, including all hotspots be taken into account. Both the incident profile and the merged profile calculated by the NLSE lack cylindrical symmetry and are thus incompatible with WAKE. Alternatively, the measured incident pulse profile could be input into a three-dimensional (3D) PIC simulation that is not restricted by cylindrical symmetry. This is not feasible here for two reasons. First, the phase profile of the incident pulse, which significantly affects its initial non-linear propagation, is not accurately known, and would thus have to be entered into a simulation as a free experimentally unknown parameter. Second, in view of the X-ray source positions shown in Fig. 3c , the simulated pulse would have to be propagated through the entire 7-cm cell length with each iteration of this parameter. The computational time and expense of this approach is prohibitive. We therefore opted to represent the incident pulse qualitatively with various cylindrically symmetric profiles that matched the experimental energy and duration and could be propagated relatively quickly using WAKE. As a crude first approximation, we represented shot ‘ a ’ by a 100-J, 160-fs incident pulse of the Gaussian profile with radius w 0 =275 μm and flat phase front. This pulse self focused to 7 × 10 19 W cm −2 at z ≈40 mm (orange dashed curve ‘G’ in Fig. 4a ) and formed a bubble, but evolved too slowly to trigger injection. On the other hand, we found that various cylindrically symmetric distortions from a Gaussian profile (maintaining the same energy and duration) resulted in faster axial intensity evolution that successfully triggered injection. Evidently, rapid bubble profile evolution, known to facilitate injection [13] , can be driven by non-Gaussian structure in the drive pulse profile. Peculiarities of non-linear self focusing of non-Gaussian beams have been observed previously in gases [35] . As an example, the solid curves in Fig. 4a show results for a third-order super-Gaussian of radius w 0 =275 μm. Super-Gaussian pulses of any order develop fine-scale transverse structure analogous to Airy rings (shown in Fig. 4b at z =30 mm) as they propagate, which evidently has a role in aiding injection similar to that of hotspots in a 3D geometry, despite differing in topology. In fact, as discussed in Methods and illustrated in Fig. 5 , if we mimic an initial array of hotspots by multiplying a super-Gaussian by an azimuthally varying function f ( r, φ ), a similar Airy ring structure develops (see curve SG-3( φ ), red squares in Fig. 4b ) when it is propagated with the NLSE code, thus establishing a connection between the super-Gaussian and a hotspot array. The third-order super-Gaussian pulse undergoes two rapid self focus/defocus cycles near the cell exit. A first electron bunch, injected in conjunction with the first self focus at ~5.8 cm ( Fig. 4a , solid blue curve), accelerated to ~2 GeV in the remaining ~1.2 cm of plasma ( Fig. 4c ), in good agreement with the observed 2 GeV peak. The average accelerating field for this bunch was 1.6 GV cm −1 , somewhat smaller than the maximum field E z ≈2 GV cm −1 estimated earlier. A refocus of the drive laser near the cell exit ( Fig. 4a ) triggered a second injection that produced a low-energy electron tail ( Fig. 4c ), in qualitative agreement with the observed tail. This scenario also captures the key observation that betatron X-rays (and thus accelerated electrons) originated near the gas cell exit (see Fig. 3c ). Finally, this simulation showed that self-injected electrons were confined within ~2 μm of the axis of the ~30 μm radius bubble (see Fig. 4c , inset), consistent with the observed sub-mrad beam divergence. In contrast, an iso-intensity contour of the self-focused laser pulse at the threshold of K -shell ionization of nitrogen (black dashed curve in Fig. 4c , inset) showed that ionization of nitrogen impurities, if present, would have produced a much broader injected profile and more divergent beam, as observed in previous experiments [6] . Similar results are obtained for other cylindrically symmetric non-Gaussian distortions of the pulse profile. Thus, although the simulations do not capture the quantitative 3D evolution of laser pulse and plasma bubble, they appear to capture the correct qualitative propagation and injection physics, as well as the four key observations noted above. 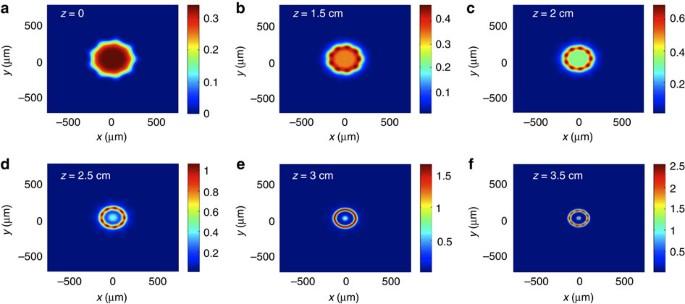Figure 5: NLSE simulation illustrating topological changes of a relativistically self-focusing laser pulse. The colour bars indicate the squared laser strength parametera2. The laser pulse evolves according to the NLSE in a plasma of densityne=5 × 1017cm−3. (a) Initial pulse atz=0 with azimuthally modulated super-Gaussian profile. Algebraic form and parameters are given in Methods. (b,c) The azimuthal perturbations quickly evolve into distinct hotspots byz=2 cm, similar to those present in the actual laser pulse. (d,e) Hotspots then evolve into a nearly cylindrically symmetric ring byz=3 cm, as the central peak intensifies. At this point, the radial profile is very similar to that of initially cylindrically symmetric super-Gaussian pulses, as shown inFig. 4b. (f) Byz=3.5 cm, the central peak becomes more intense than the outer ring. WAKE simulations of similar profiles suggest that this central peak continues intensifying rapidly, eventually forming a rapidly evolving bubble into which surrounding plasma electrons inject. Atz=3.5 cm, however, the density perturbation has already become substantial, invalidating further description by the NLSE. Figure 5: NLSE simulation illustrating topological changes of a relativistically self-focusing laser pulse. The colour bars indicate the squared laser strength parameter a 2 . The laser pulse evolves according to the NLSE in a plasma of density n e =5 × 10 17 cm −3 . ( a ) Initial pulse at z =0 with azimuthally modulated super-Gaussian profile. Algebraic form and parameters are given in Methods. ( b , c ) The azimuthal perturbations quickly evolve into distinct hotspots by z =2 cm, similar to those present in the actual laser pulse. ( d , e ) Hotspots then evolve into a nearly cylindrically symmetric ring by z =3 cm, as the central peak intensifies. At this point, the radial profile is very similar to that of initially cylindrically symmetric super-Gaussian pulses, as shown in Fig. 4b . ( f ) By z =3.5 cm, the central peak becomes more intense than the outer ring. WAKE simulations of similar profiles suggest that this central peak continues intensifying rapidly, eventually forming a rapidly evolving bubble into which surrounding plasma electrons inject. At z =3.5 cm, however, the density perturbation has already become substantial, invalidating further description by the NLSE. Full size image In summary, we have demonstrated self-injected quasi-monoenergetic LPA of electrons well beyond 1 GeV in a range of plasma density (3≤ n e ≤6 × 10 17 cm −3 ) significantly lower than previous quasi-monoenergetic LPA experiments. LPAs at these densities are required for table-top X-ray free electron lasers [10] and to achieve the ~10 GeV stage envisioned [9] for a future laser-driven collider. Although quasi-monoenergetic acceleration to 2 GeV with unprecedented divergence ( θ e ~0.5 mrad) and excellent pointing stability (1.4 mrad r.m.s.) is reported here, significant improvements in peak electron energy and beam quality appear feasible with better laser-pulse quality to increase self-guiding length, and specialized injection techniques [19] , [22] , [24] , [25] to reduce dark current and energy spread. Laser The Texas Petawatt Laser uses optical parametric chirped pulse amplification followed by chirped pulse amplification in two different types of neodymium-doped glass [26] . At full power, it can produce 1.1 PW (170 J, 150 fs FWHM) laser pulses at centre wavelength 1.057 μm, approximately once per hour. A spherical mirror tilted 1° off axis focused the pulse near the gas cell entrance. Estimated focused profiles (for example, Fig. 4a ) were obtained by imaging equivalently focused light that was leaked through a high-reflectance mirror upstream of the focusing mirror. These images do not account for possible influence of laser-pulse interaction with the gas plume emanating from the cell entrance aperture. An electronic trigger pulse from the laser timing system initiated filling of the gas cell ~4 ms before the laser-pulse arrival. A calibrated fast pressure transducer (Measurement Specialties Model EPET21-0.13B-/M/Z2/V05/L02F) measured He pressure versus time, and also recorded an acoustic shock when the laser pulse arrived ( Fig. 1g ), enabling determination of gas pressure, and thus plasma density n e , during the laser-plasma interaction with ±10% accuracy. Electron energy measurement As the dispersion of the magnet was relatively small for GeV electron energies, special care was taken to assure accurate energy measurement. We followed the basic ‘two-screen’ method of Clayton et al. [6] and Pollock et al. [30] , in which electron energies and launch angles were determined uniquely for each shot by calculating electron trajectories that passed through three measured reference points (source, fiducial marker and fiducial shadow). However, we made several improvements to achieve unprecedented resolution. First, the initial screen of Clayton et al. [6] and Pollock et al. [30] was replaced with two rows of 127 μm diameter tungsten fiducial wires that cast shadows in both X-ray and dispersed electron signals. These wires and their shadows were much more sharply defined and precisely positioned than intrinsic electron spectral features used previously [6] , [30] , thereby defining two of the required reference points more precisely. Fiducial wires and IP detectors were mounted in precisely machined frames, mounted in turn on a machined plate inside the vacuum chamber, reducing uncertainty in their lateral positions to ±25 μm. The IP scanner (Fuji FLA-7000) was calibrated spatially by scanning an IP irradiated with a radioactive source through a machined grid of holes in a metal plate. Wire diameter was chosen based on GEANT4 (ref. 36 ) absorption and scattering simulations, which showed that despite negligible absorption of GeV electrons, scattering produced high-contrast shadows that were sharply bounded because of low beam divergence. Use of discrete wires rather than a continuous screen also avoided unwanted scatter of electrons passing between fiducial markers. Electron scattering in the 75-μm thick aluminium laser beam deflector slightly reduced contrast, but did not significantly affect determination of shadow positions to within ±1/2 pixel (±50 μm) on the IPs. Second, we took advantage of the high-contrast, sharply bounded shadows that the fiducial wire arrays cast independently in the betatron X-ray signals, which GEANT4 simulations showed were caused primarily by absorption. As the angular spread of the X-rays was wide enough that they cast shadows of two or more fiducial wires, and as X-rays do not bend in the magnetic field, conventional triangulation based on these X-ray shadows enabled the third reference point (source position) also to be localized more precisely (±75 μm transversely, ±1 cm longitudinally) than in previous works [6] , [30] . Determining this X-ray source point was the first step in electron energy analysis. This X-ray source point was then assumed to coincide with the electron source. As a second step, shadows in the electron spectra were analysed using calculated electron trajectories constrained to pass through this source point, a fiducial wire and its shadow. These constraints unambiguously determined the electron energy and launch angle of electron trajectories that passed through each fiducial wire. Third, our total trajectory length (2.7 m) was larger than in previous work, further aiding accuracy. The small size of fiducial wires and shadows, combined with precise positioning of components, and accurate determination of X-ray and electron shadow positions, enabled precise recovery of energy-dependent electron trajectories, including launch angle. As a cross-check, we confirmed that electron launch angles were nearly energy independent for shots that produced electron signals with negligible energy-dependent vertical angle displacements. The electron bunch divergence (0.5 mrad FWHM) together with uncertainties in fiducial and shadow positions yielded an electron spectrometer resolution of ±100 MeV (±5%) at 2 GeV at the 2σ error level for the shots shown in this paper. Electron detection and charge measurement Charge was determined by independently calibrating electron signals obtained from IPs and a LANEX phosphor screen. To determine charge from IPs, independent measurements were performed using high-sensitivity (Fujifilm BAS-IP MS 2040, 100 μm pixels) and high-resolution (BAS-IP SR 2040, 50 μm pixels) IPs. Photo-stimulated luminescence (PSL) levels of the IPs were determined using a Fuji-labelled FLA-7000 IP scanner. Repeated scans were performed to reduce and finally remove saturation when it was present; a saturation factor was then computed by comparing the PSL drop between the first and the last scan for commensurate unsaturated regions in the two scans; this factor was applied to the PSL from the unsaturated image. To convert PSL to charge, weighted fits to published sensitivity (PSL/electron) measurements [37] , [38] , [39] yielded sensitivity as a function of energy. Light from the LANEX phosphor screen and the plastic scintillator (ELJEN Technology, EJ-200) were focused onto a colour charge-coupled device (CCD) camera (Basler, scA 1600-14fc). LANEX and scintillator images were distinguished by their different colours. The CCD output at the LANEX phosphorescence wavelength was related to the charge exciting the LANEX using the published emission spectrum and absolute calibration for Kodak LANEX Regular [40] , in conjunction with the measured CCD quantum efficiencies. Betatron X-ray detection and analysis Betatron X-rays were detected on IP HS and their spectrum derived from the signal transmitted through Al and Cu filter packs. The latter was normalized to the incident intensity profile, reconstructed from the signal transmitted through gaps in the filter. To extract the X-ray spectrum, we followed the method of Ta Phuoc et al. [41] Assuming a sufficiently narrow form of the function f k ( ω )=( T k ( ω )− T k +1 ( ω )) R ( ω )/(10 −3 ω ), where T k is the transmittance of filter k and R is the IP response in units of PSL/photon, the number of photons per 0.1% bandwidth, assigned to the mean of the distribution f k ( ω ), is (10 −3 ω dN γ / d ( ω )] ω k =( S k — S k +1 )/∫ d ( ω ) f k ( ω ), where S k is the signal transmitted by filter k . To obtain a lower bound on photon number, total PSL was divided by the IP sensitivity (~0.0092 PSL per photon) at the photon energy (18 keV) at which IP HS is most sensitive. Simulations Simulations of laser-pulse propagation and plasma wave dynamics were performed using WAKE [34] , a fully relativistic PIC code in axisymmetric geometry. WAKE calculates the quasi-static plasma response to the ponderomotive force averaged over the laser period and to the self-consistent electromagnetic fields of the plasma wake. Propagation of the laser beam is described in the extended paraxial approximation with group velocity dispersion taken into account. Electron self injection and acceleration were modelled using test particles not subject to the quasi-static assumption, a valid approach in the limit of low-injected charge where the effects of beam loading are not significant [13] . For illustrative calculations of the initial propagation of non-axisymmetric pulses, we numerically solved the NLSE where γ' =(1+ a 2 /2) 1/2 is the Lorentz factor of plasma electrons in the laser field, and k and k p are the laser and plasma wave numbers, respectively. We verified that the NLSE accurately reproduced results of WAKE as long as fractional density perturbations were small. However, the NLSE does not properly model finite pulse duration and bubble formation. Thus, we used it for the limited purpose of illustrating how laser pulses with hotspots, represented by initial azimuthally varying super-Gaussian envelopes of the form , where m and n are integers and α a fraction between 0 and 1, change in topology as they begin to self focus. As an example, Fig. 5 illustrates how a pulse initially with m =9, n =6, α =0.25, a 0 =0.58 and w 0 =275 μm evolves in the transverse x — y plane when it propagates through plasma of density n e =5 × 10 17 cm −3 (that is, P / P c ≈20). Distinct hotspots evident early in the propagation ( z ≤2 cm) evolve into a nearly azimuthally symmetric Airy-like ring by z ~3 cm, as the central peak intensifies. As shown in Fig. 4b , the resulting radial profile closely resembles those obtained with initially cylindrically symmetric super-Gaussian pulses that were correlated with rapid axial intensity evolution and electron self injection. How to cite this article: Wang, X. et al. Quasi-monoenergetic laser-plasma acceleration of electrons to 2 GeV . Nat Commun. 4:1988 doi: 10.1038/ncomms2988 (2013).